The role of random nanostructures for the omnidirectional anti-reflection properties of the glasswing butterfly The glasswing butterfly ( Greta oto ) has, as its name suggests, transparent wings with remarkable low haze and reflectance over the whole visible spectral range even for large view angles of 80°. This omnidirectional anti-reflection behaviour is caused by small nanopillars covering the transparent regions of its wings. In difference to other anti-reflection coatings found in nature, these pillars are irregularly arranged and feature a random height and width distribution. Here we simulate the optical properties with the effective medium theory and transfer matrix method and show that the random height distribution of pillars significantly reduces the reflection not only for normal incidence but also for high view angles. Camouflage by transparency requires low absorption and reflection as well as low scattering of light. These constraints are hard to fulfil for terrestrial plants and animals for several reasons [1] . First, the large difference between the refractive indices of living tissues ( n =1.3–1.55) and air ( n =1) results in significant surface reflections. Second, most terrestrial organisms require pigmentation to protect themselves against the comparably high levels of ultraviolet radiation on land. Finally, as buoyant forces are absent on land, supporting anatomical structures are needed and they are often opaque. Consequently, transparency is uncommon for terrestrial organisms but it is frequently found in aquatic life where the higher refractive index of water ( n =1.33) decreases the refractive index contrast [1] . The wings of the butterfly Greta oto ( Fig. 1a ) are an interesting example for transparency on land [1] , [2] . It is an Ithomiini tribe member living in Central America and the transparent parts of its wings make it difficult for predatory birds to track the butterfly during the flight [3] . In a recent study [2] , it was suggested that the high transparency might be caused by the hexagonal packing of microscopic nipples. Indeed, even sized and hexagonally packed nipples serve as anti-reflection surfaces in moth eyes [4] , hawk moth wings [5] and cicada wings [6] , [7] . However, similar to the wax structures found on the wing membrane of the dragonfly Aeshna cyanea [8] , the microscopic structures in the transparent parts of the wings of Greta oto are far from being regular. The transparent parts of glasswings are covered with randomly sized nanopillars of high aspect ratio. Interestingly, the scatter of height and width of these pillars is the origin of the omnidirectional anti-reflection properties of the glasswing butterfly. 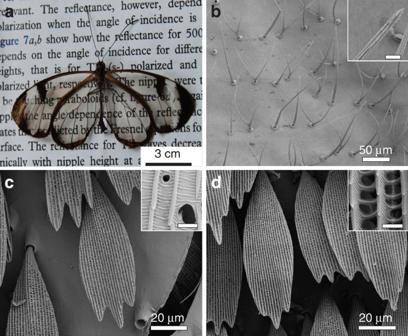Figure 1: The glasswing butterfly and its scales. (a) Photo of a glasswing butterfly (Greta oto). Its wings feature three regions—transparent, dark brown and white. (The text behind the butterfly is page 664 from ref.22). (b) The SEM image of the transparent region reveals that this part of the wing is covered with ≈2 μm thick and ≈40 μm long bristles or microhairs (see inset). The areas between these microhairs are covered with nanopillars that are analysed in detail inFig. 2. Scales found in the brown (c) and white regions (d) look quite similar at first sight but the brown scales have membranes between their ridges, while the white ones do not (see corresponding insets). The length of the scale bars in the insets is (b) 4 μm and (c,d) 1 μm. Figure 1: The glasswing butterfly and its scales. ( a ) Photo of a glasswing butterfly ( Greta oto ). Its wings feature three regions—transparent, dark brown and white. (The text behind the butterfly is page 664 from ref. 22 ). ( b ) The SEM image of the transparent region reveals that this part of the wing is covered with ≈2 μm thick and ≈40 μm long bristles or microhairs (see inset). The areas between these microhairs are covered with nanopillars that are analysed in detail in Fig. 2 . Scales found in the brown ( c ) and white regions ( d ) look quite similar at first sight but the brown scales have membranes between their ridges, while the white ones do not (see corresponding insets). The length of the scale bars in the insets is ( b ) 4 μm and ( c , d ) 1 μm. Full size image Here we analyse the specular and diffuse reflection of the glasswing and explain the concept of transparency by randomness. Angle-resolved spectroscopy reveals that the transparent parts of the glasswing have a low specular reflection of 2% (two air/wing interfaces) in the visible regime for high radiation angles of 65° and close to 5% for incidence angles of 80°. We simulate these omnidirectional anti-reflection properties by considering a Gaussian height distribution of the nanopillars as in the glasswing. By varying the size and distribution of the structures, we demonstrate that the randomness is the origin of the remarkable broadband and omnidirectional anti-reflective property of Greta oto . Experimental analysis of the glasswing butterfly The wings of the Greta oto butterfly feature dark brown, white and transparent regions. Frequently, the brown regions appear in an orange–brown colour. The scales found in these three distinguished regions are compared in Fig. 1 by scanning electron microscopy (SEM) images. The transparent region is covered with high aspect ratio microhairs that are generally known as piliform scales or bristles [9] , [10] . The hairs are 40–50 μm apart from each other and their typical thickness and height are about 2 and 40 μm, respectively. These specialized setae/bristle shapes occur in several Lepidopteran and are commonly believed to serve for defensive purposes [11] . Furthermore, the microhairs improve the hydrophobicity of the wings [12] . The SEM images of the brown and white scales show the common oval shape with a typical width of 50 μm and length of 200 μm (refs 9 , 11 ). The feature of interest for our study, however, is found on the thin wing membrane, which we analysed by SEM. The top view ( Fig. 2a ) displays the irregular positioning of the nanopillars. The two-dimensional Fourier power spectrum of the top view SEM image of the nanostructures shows a ring-shaped distribution of the squared Fourier components ( Fig. 2b ) caused by the disordered arrangement of nanopillars. Nevertheless, the finite diameter of the ring indicates an average characteristic distance of the pillars in the range of 100–140 nm, which is lower than the wavelengths considered in this study (that is, <200 nm). Interestingly, the randomness of the nanopillar distribution is not only limited to their arrangement. The tilted view in Fig. 2c reveals the random height of the nanopillars. These fine pillars stand on top of pedestals with a cone-like shape and a typical height of 160–200 nm as revealed by the high-resolution image in Fig. 2d . Examining the dorsal and ventral sides of the transparent parts of the wings, we observed no differences in their structure ( Supplementary Fig. 1 ). Furthermore, we cut the wing membrane in the transparent region with a focused ion beam (FIB). Its thickness is about 550 nm and no special features were found in the cross-section ( Fig. 2e ). To quantify the randomness of the nanopillars, we determined the characteristic dimensions of the nanopillars by electron microscopy on the transparent region of the dorsal wing. The radii of the nanopillars were measured at the intersection of pedestals and pillars. Height and radius of the pillars scatter and typical values are between 400–600 nm and 40–60 nm, respectively. Consequently, the typical aspect ratio is about 5. Some nanopillars, however, reach an aspect ratio of 10. The histogram of the height analysis is shown in Fig. 2f and it can be approximated by a Gaussian distribution with a variance of σ h =100 nm. Also the position of the pillars scatters and the average distance between the pillars is d =120±20 nm (centre to centre), which is in agreement with the fast Fourier transform analysis. 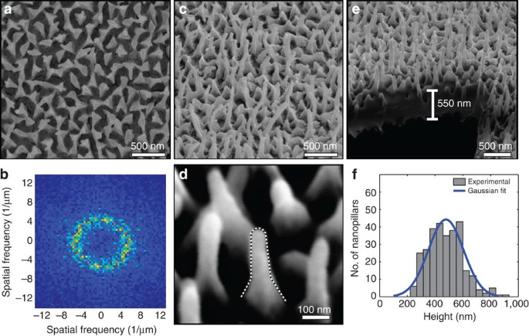Figure 2: Anti-reflective nanostructures of the glasswing. These structures are found in the transparent regions of the wings between the microhairs (seeFig. 1). The top view (a) shows the quasi-random positioning of the pillars that is confirmed by the two-dimensional Fourier power spectrum of the position of the nanostructures, which is calculated from this SEM image and shown inb. The tilted view (c) reveals the random height and width distribution of the high aspect ratio nanopillars. (d) A high-resolution image clarifies their shape, which is modelled later as a thin pillar with cone shaped pedestal. (e) A cross-section of the wing membrane was prepared by FIB and imaged by SEM. No internal features were observed in the thin base membrane. (f) Statistical analysis of the nanopillars height measured on the dorsal side of a transparent region of a glasswing. The histogram shows the height distribution of the nanopillars. A Gaussian profile with a mean height ofand a variance ofσh=100 nm describes the experimental data. Figure 2: Anti-reflective nanostructures of the glasswing. These structures are found in the transparent regions of the wings between the microhairs (see Fig. 1 ). The top view ( a ) shows the quasi-random positioning of the pillars that is confirmed by the two-dimensional Fourier power spectrum of the position of the nanostructures, which is calculated from this SEM image and shown in b . The tilted view ( c ) reveals the random height and width distribution of the high aspect ratio nanopillars. ( d ) A high-resolution image clarifies their shape, which is modelled later as a thin pillar with cone shaped pedestal. ( e ) A cross-section of the wing membrane was prepared by FIB and imaged by SEM. No internal features were observed in the thin base membrane. ( f ) Statistical analysis of the nanopillars height measured on the dorsal side of a transparent region of a glasswing. The histogram shows the height distribution of the nanopillars. A Gaussian profile with a mean height of and a variance of σ h =100 nm describes the experimental data. Full size image To understand the origin of the anti-reflection properties of the glasswing butterfly, we have to prove that they originate from the microscopic (the nanopillars) and not from macroscopic features (the bristles or microhairs). To reveal any optical effect of the microhairs on the reflection, we removed them by gently pressing the adhesive tape to the wing and stripping it carefully. Afterwards, we analysed this sample with an optical spectrometer (ultraviolet–visible Spectrometer Lambda 1050, PerkinElmer Inc.). SEM images of the bristle-free wing sample showed no harm to the nanopillars and corresponding diffusive reflection spectra of the transparent wing area with and without hair overlapped ( Supplementary Fig. 2 ). Therefore, it is evident that the micrometre-sized hairs do not play any role in the transparency of the glasswing. As the structures on the dorsal and ventral sides are alike ( Supplementary Fig. 1 ), it is comprehensible that both sides of the wing have the same reflective properties. This is confirmed by the optical spectra shown in Fig. 3a . The total reflection is remarkably low in the visible regime. In comparison with the bare glass, which is known to reflect about 8% of light under normal incidence (two surfaces [13] ), the glasswing reflection of 2% (two surfaces) in the visible regime is about four times lower while their refractive indices are quite close [14] , [15] , [16] . The low reflection is also observed for wavelengths in the ultraviolet to near infrared (NIR) regime. The forward scattering measurement shown in the inset of Fig. 3a verifies the low scattering of the transparent parts of the glasswing. The transmittance drops down from 84% to almost 0% within a scattering angle of 5°. 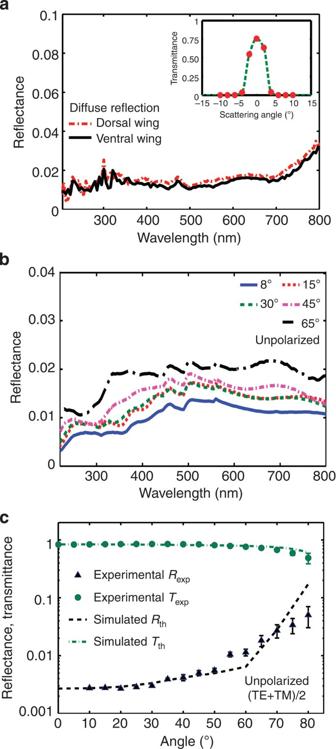Figure 3: Experimental reflectance spectra of the transparent region of the glasswing butterfly. (a) The diffuse reflection measured in the transparent areas on the dorsal and ventral wing is comparable within the experimental uncertainty. Reflection values are about 2% (two surfaces) for wavelengths between 390 and 700 nm and increase up to 3% for 800 nm. The forward scattering measurement, recorded for a wavelength of 633 nm and shown in the inset, proofs the low haze of the glasswing. (b) The omnidirectional and broadband anti-reflection is observed for all visible wavelengths. The angle-resolved specular reflection measured on the transparent dorsal wing region from 8° to 65° reveals that the reflection is below 2.2% even for angles up to 65°. (c) The triangles show the angle-dependent reflection measured with an unpolarized focused laser light with 632.8 nm wavelength (errors bars correspond to the estimated experimental error). This result proves that the overall reflection properties of the glasswing are present even for angles up to 80°. The circles display the angle-resolved transmission recorded with an unpolarized 633 nm light source. The dashed black line and the green dashed-dotted line are calculated with the presented glasswing model of nanopillars with pedestals taking into the account the reflection on the backside of the membrane. Figure 3: Experimental reflectance spectra of the transparent region of the glasswing butterfly. ( a ) The diffuse reflection measured in the transparent areas on the dorsal and ventral wing is comparable within the experimental uncertainty. Reflection values are about 2% (two surfaces) for wavelengths between 390 and 700 nm and increase up to 3% for 800 nm. The forward scattering measurement, recorded for a wavelength of 633 nm and shown in the inset, proofs the low haze of the glasswing. ( b ) The omnidirectional and broadband anti-reflection is observed for all visible wavelengths. The angle-resolved specular reflection measured on the transparent dorsal wing region from 8° to 65° reveals that the reflection is below 2.2% even for angles up to 65°. ( c ) The triangles show the angle-dependent reflection measured with an unpolarized focused laser light with 632.8 nm wavelength (errors bars correspond to the estimated experimental error). This result proves that the overall reflection properties of the glasswing are present even for angles up to 80°. The circles display the angle-resolved transmission recorded with an unpolarized 633 nm light source. The dashed black line and the green dashed-dotted line are calculated with the presented glasswing model of nanopillars with pedestals taking into the account the reflection on the backside of the membrane. Full size image Angle-resolved spectra of specular reflection recorded for the wavelength regime of 200–800 nm are plotted in Fig. 3b for unpolarized light (ultraviolet–visible Spectrometer Lambda 1050, PerkinElmer Inc.). The overall reflection slightly increases with the angle of incidence. A reflection of up to 2.2% is observed for an angle of 65°, while all the values are well below 2% for lower angles. However, due to the comparable large spot size (4 × 4 mm 2 ) and technical constraints of this set-up for high-angle measurements, we use a home-built focused laser-based angle-resolved reflectance spectroscope with an unpolarized laser light of 632.8 nm wavelength [17] . In this way, we are able to exclude the parasitic absorption on the veins of the Glasswing from the measurement because the spot size of this set-up is only 50 μm in diameter and can be easily focused on the transparent wing parts between the veins. As shown by the triangles in Fig. 3c , only 0.2% of reflection is measured for a normal angle of incidence in this case and a low reflection of 5% is measured even for a large angle of 80°, which reveals the high omnidirectional anti-reflective performance of the transparent region of the glasswing. In addition, we measured the transmittance of the transparent parts of the glasswing via transmission geometry (Cary 5000 ultraviolet–visible–NIR spectrophotometer, Agilent Technologies Inc.). The circles in Fig. 3c show that the transmission is close to 84% for a wavelength of 633 nm and decreases only slightly for high angles. This result verifies the omnidirectional high transparency of the glasswing. At first sight, one is tempted to compare the remarkably low reflection of the glasswing with the structure of nipples found in the moth eye [2] . According to the famous study of Bernhard and Miller [18] in the 1960s, the index of refraction changes gradually in the moth eye due to submicroscopic nipples, and such structuring reduces the reflection of light. In the meantime, this principle has been also found in eyes [19] and wings [5] , [6] of other insects, and can be applied for the fabrication of biomimetic artificial anti-reflection coatings [20] , [21] . All these nipple structures, however, feature a highly periodic distribution with constant height and aspect ratios of 1 to 2. The nanopillars of the glasswing, on the other hand, are highly random in size and have much higher aspect ratios up to 10. As shown by the following theoretical analysis, this structural scatter is the key to the high omnidirectional anti-reflection properties of the glasswing butterfly. Optical modelling of the reflection of glasswings To analyse the anti-reflection properties of the glasswing, we simulate the optical properties of its nanostructure with an analytical approach. It explicitly considers the random height distribution of the nanopillars. We start with the calculation of the effective volume fraction f ( z ) of the wing material similar to the previous studies of gradient refractive index anti-reflective structures [20] , [21] , [22] . The subsequent application of the effective medium theory [23] , [24] allows the calculation of the refractive index profile of the random nanopillars. Afterwards, the transfer matrix method (also known as the multilayer model) [20] , [22] , [24] , [25] enables us to compute the reflection and transmission for a given polarization and for all angles of incidence. In the following, we introduce two shapes to model the nanopillars found in the transparent parts of the glasswing ( Fig. 4a ). First, we simplify these structures ( Fig. 2d ) as cylindrical nanopillars with constant radius but consider a Gaussian height distribution ( Fig. 4a ). We assume a hexagonal unit cell with an area of where d is the centre to centre distance to the next nanopillar. Therefore, the area of a nanopillar is constant throughout its height, that is, , but the height distribution of the cylinders is random. From the experimental analysis in Fig. 2f , it follows that the height of the nanopillars can be roughly described by a Gaussian distribution. The origin of the z axis is defined to be at the base of the nanopillars. Consequently, the probability of finding a cylinder of height h at position z is given by the normal distribution . 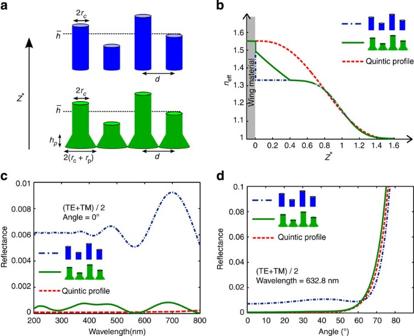Figure 4: Simulation of the anti-reflection properties. (a) Schematics of the analysed anti-reflection structures (not to scale). The glasswing structure is modelled by nanopillars with fixed radius but randomly distributed height (blue, top). This model of random nanopillars is greatly improved if we consider also the pedestals of the glasswing structures by adding pedestals of heighthp(green, bottom). (b) Profiles of the effective refractive index (neff) for three different topologies. Starting from the wing membrane, the refractive index for the model of random nanopillars (blue dashed-dotted line) is nearly constant before it decreases smoothly tonair. The plateau disappears if we add the pedestals to the nanopillars. In this case, the refractive index decreases nearly linearly before it decreases smoothly (solid green line). The profiles are compared with a quintic profile (red dashed line). (c) Optical modelling of the different models considering unpolarized light, that is, averaging the s(TE)- and p(TM)-polarizations. Reflection spectra of random nanopillars with and without pedestals are compared with a quintic profile for normal incidence. The nanopillars of random height on top of pedestals show better anti-reflection properties compared with the one without pedestals. (d) Reflection as a function of the incidence angle for incoming unpolarized light with a wavelength of 632.8 nm. The random nanopillars with Gaussian distribution provide similar behaviour as of the quintic profile in terms of omnidirectional anti-reflection properties. With this assumption, we can average over all nanopillars and get the volume fraction of the nanopillars Figure 4: Simulation of the anti-reflection properties. ( a ) Schematics of the analysed anti-reflection structures (not to scale). The glasswing structure is modelled by nanopillars with fixed radius but randomly distributed height (blue, top). This model of random nanopillars is greatly improved if we consider also the pedestals of the glasswing structures by adding pedestals of height h p (green, bottom). ( b ) Profiles of the effective refractive index ( n eff ) for three different topologies. Starting from the wing membrane, the refractive index for the model of random nanopillars (blue dashed-dotted line) is nearly constant before it decreases smoothly to n air . The plateau disappears if we add the pedestals to the nanopillars. In this case, the refractive index decreases nearly linearly before it decreases smoothly (solid green line). The profiles are compared with a quintic profile (red dashed line). ( c ) Optical modelling of the different models considering unpolarized light, that is, averaging the s(TE)- and p(TM)-polarizations. Reflection spectra of random nanopillars with and without pedestals are compared with a quintic profile for normal incidence. The nanopillars of random height on top of pedestals show better anti-reflection properties compared with the one without pedestals. ( d ) Reflection as a function of the incidence angle for incoming unpolarized light with a wavelength of 632.8 nm. The random nanopillars with Gaussian distribution provide similar behaviour as of the quintic profile in terms of omnidirectional anti-reflection properties. Full size image where is the complementary error function. The remaining fraction of air is given by f air ( z )=1– f pillars ( z ). After determining the volume fraction, the effective refractive index n eff can be calculated for any z using the well-known Maxwell–Garnett model [20] , [23] , [24] where n eff , n chitin and n air are the refractive indices of the mixture, chitin and air, respectively. For an easy comparison of different models and shapes, we use normalized scaling in the following. We assume a typical refractive index of chitin and air without absorption as n chitin =1.57 [14–16] and n air =1, respectively. The dash-dotted line in Fig. 4b represents the effective refractive index calculated for the model of nanopillars with random heights (equation (1)). Here we considered typical parameters corresponding to the values observed in the SEM analysis in Fig. 2 , that is, , σ h =100 nm, d =120 nm and r c =50 nm. The increase of the effective refractive index from air to wing material is smooth due to the random height distribution of the nanopillars. This shape resembles the form of a quintic profile, which is close to the optimum profile for a graded-index anti-reflection coating [26] , [27] , [28] . To compare it with our model of random nanopillars profiles, we added a quintic profile with a height h max =800 nm (red dashed line) to Fig. 4b . Indeed, the quintic profile matches the glasswing model perfectly in the air/nanopillar region for the chosen parameters. However, for lower z * values, the refractive index of the random nanopillars reaches a plateau and is nearly constant. Therefore, it differs from the quintic profile in the nanopillar/membrane region. From these effective refractive indices, we computed the reflection spectra for s-polarization (electric field is normal to the plane of incidence, TE) and p-polarization (electric field is parallel to the plane of incidence, TM). Furthermore, we calculate the reflection for different angles of incidence applying the multilayer model. For that, the structure is divided into 1,000 thin horizontal layers and the refractive index of each layer is calculated using the effective medium theory. Afterwards, the optical admittance and the corresponding reflection spectra of the stack of thin layers are calculated using the characteristic matrix method (see refs 20 , 21 , 24 and references therein for more details). The reflection spectrum under normal incidence plotted in Fig. 4c as a function of the wavelength for the model of random nanopillars (dashed-dotted line) and the quintic profile (dashed line). The reflection is well below 1% (one surface) for both cases and all wavelengths. The reflection of the quintic profile, however, is considerably lower as for the nanopillars (≈0.03%). Nonetheless, this simple model of random nanopillars with Gaussian height distribution already has good omnidirectional anti-reflection properties as demonstrated by the comparison in Fig. 4d where we plotted the reflection versus incidence angle. Here the reflection stays nearly constant till it increases for larger angles. Interestingly, the random nanopillars are slightly better as the quintic profile for high angles and reflect less light for angles larger than 65° and for the chosen parameters. This omnidirectional broadband anti-reflective properties become even better and almost equal to the ones obtained with the quintic profile, if the model of the glasswing nanostructures is further improved by considering also pedestals observed in the SEM images ( Fig. 2c ). Figure 4a shows a schematic of the assumed structure where we added cone-like pedestals of height h p . These pedestals increase the radius at the bottom of the glasswing structures to r = r c +r p . At the height h p , the radius decreases to r = r c . For this pedestal shape, the volume fraction of the glasswing is given by For r p , h p →0, this equation converges to the model of random nanopillars (equation (1)). With the consideration of the pedestals (green solid line in Fig. 4b ), the refractive index in the region of the pedestals comes closer to the quintic profile and the plateau of the random nanopillars disappears. Consequently, the overall reflection behaviour is improved and approaches that of the quintic profile. The reflection of this glasswing model (green solid line in Fig. 4b ) is now ∼ 0.05% for all wavelengths and much lower than for the simple model of random nanopillars. However, the omnidirectional anti-reflection behaviour is nearly as good as for the quintic profile. The comparison of the two cases in Fig. 4 shows that both the curves nearly overlap and that the reflection is below 5% for angles up to 70°. For any type of pedestals we added to the random nanopillars, we observed an improvement of the omnidirectional anti-reflection properties ( Supplementary Fig. 3 ). Any shape of pedestals that converges the plateau of the effective refractive index of the random nanopillars towards the quintic profile shows this effect. To compare the advanced glasswing model with the experimental results, we have to additionally consider the absorption by the membrane and take into account the multiple reflections of light on its backside. Since the wing membrane is surrounded by nanopillars and air from two sides and there is almost no scattering, we adapt the reflection and transmission equations from ref. 29 . More details of the calculation are provided in the Supplementary Material . We varied all structural parameters of the pedestals ( r p , h p , σ h ) and the extinction coefficient κ . The best fit was obtained for κ =0.007±0.001, which is close to previously reported values [8] . The dashed and dash-dotted line in Fig. 3c are fits of the simulated transmission and reflection to the experimental data for r p =6 nm, h p =170 nm and σ h =135 nm. The pedestals do not touch for this radius. The simulated reflection and transmission are in agreement with the experimental data. For angles higher than 70°, however, the measured data even outperforms simulations. We contribute this deviation to possible experimental uncertainties and effects not considered in our simulation so far (non-uniform thickness and uneven surface of the membrane, possible overlaps to brown veins due to expanded laser spot size for very high angles). Nonetheless, this result proofs that the model of nanopillars with pedestals describes correctly the overall omnidirectional anti-reflection properties of the glasswing. Finally, we discuss how three significant parameters of the advanced glasswing model—the random height of the nanopillars and the width and height of the pedestals—influence the anti-reflection behaviour. We do that by systematically varying the magnitude of the different parameters. As in the simulations of Fig. 4 , we do not consider absorption for these exemplary calculations. First, we change the ‘randomness’ of the nanopillars via the variance σ h . As depicted in Fig. 5a , the refractive index profile becomes smoother if the variance is increased. This feature significantly improves the omnidirectional anti-reflection feature. For a comparably large value of σ h =150 nm, the reflection is lower than 10% for angles below 80°. Consequently, it is favourable to increase the variance to obtain better anti-reflection properties. The variance, however, is limited for a given average height of the nanopillars. By decreasing the variance to 50 nm, the reflection increases to 30% for 80°, which is three times higher than for the highest variance value. For a non-random structure with zero variance (dashed line), all nanopillars have the same height and the omnidirectional anti-reflection property is nearly lost. Nonetheless, the reflection at normal incidence is below 2.5%. As second parameter, we change the radius of the cone-like pedestals from 0 nm to the maximum possible value of r p = d /2– r c =10 nm. As shown in Fig. 5b , the steepness of the effective refractive index profile between the plateau and the wing membrane depends directly on r p . The pedestal radius affects mainly the reflection value for low angles but decreases only slightly the reflection for large angles above 65°. A similar effect is observed with the change of the height of the pedestals. As shown in Fig. 5c , a decrease of the pedestals height increases the reflection for low angles, while it is slightly decreased for high angles. Therefore, to obtain the best omnidirectional anti-reflective properties, width and height of the pedestals have to be optimized. At the same time, larger pedestals increase the mechanical stability of the nanopillars. Interestingly, the glasswing pedestals seem to be optimized in such a way. The shape of the pedestals changes the reflectance properties only slightly ( Supplementary Fig. 3 ). Consequently, the pedestals improve the overall anti-reflection behaviour, while the randomness is the key factor for the unique broadband, omnidirectional anti-reflection properties of the glasswing. 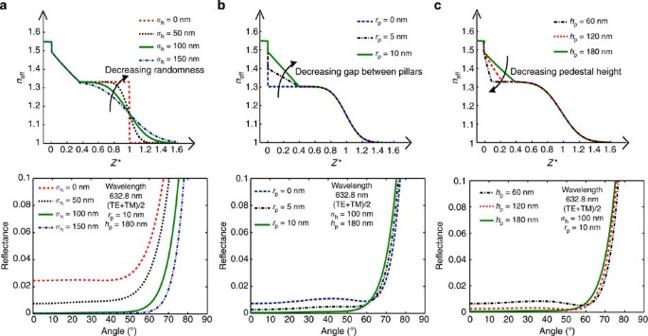Figure 5: Parameter variation of the optical model. (a) The varianceσhstrongly influences the shape of the effective refractive index profile near its turning point atz*=1. The smaller the variance the steeper is the increase of the refractive index towards the wing membrane. Forσh=0 nm, it is a step function. The omnidirectional anti-reflection properties of the extended glasswing model strongly depend on the variance of the Gaussian distribution. Keeping all the other parameters fixed, the angle-dependent reflection is calculated varying the s.d. (σh) for unpolarized light with a wavelength of 632.8 nm. Reflection is the highest forσh=0 nm (red dashed line) and decreases if the variance is increased to 50 nm (black dotted line), 100 nm (green solid line) and 150 nm (blue dash-dotted line). (b) Influence of the pedestals’ size on the reflection can be observed if their size is increased from 0 nm to the maximum possible value of 10 nm. In this way, the gap at the bottom of the pillars disappears and therefore, the plateau of the effective refractive index near the wing vanishes. The best anti-reflection behaviour is observed when the pedestals touch each other, that is, forrp=10 nm. However, this comes along with a more angle-sensitive behaviour for angles above 65°. (c) The effective refractive index profile of the nanopillars changes with the pedestals height which is decreased from 180 to 60 nm. For lower angles, the reflection decreases with the height of the pedestals. For larger angles (>60°), however, the anti-reflection is slightly better for smaller pedestals. Figure 5: Parameter variation of the optical model. ( a ) The variance σ h strongly influences the shape of the effective refractive index profile near its turning point at z *=1. The smaller the variance the steeper is the increase of the refractive index towards the wing membrane. For σ h =0 nm, it is a step function. The omnidirectional anti-reflection properties of the extended glasswing model strongly depend on the variance of the Gaussian distribution. Keeping all the other parameters fixed, the angle-dependent reflection is calculated varying the s.d. ( σ h ) for unpolarized light with a wavelength of 632.8 nm. Reflection is the highest for σ h =0 nm (red dashed line) and decreases if the variance is increased to 50 nm (black dotted line), 100 nm (green solid line) and 150 nm (blue dash-dotted line). ( b ) Influence of the pedestals’ size on the reflection can be observed if their size is increased from 0 nm to the maximum possible value of 10 nm. In this way, the gap at the bottom of the pillars disappears and therefore, the plateau of the effective refractive index near the wing vanishes. The best anti-reflection behaviour is observed when the pedestals touch each other, that is, for r p =10 nm. However, this comes along with a more angle-sensitive behaviour for angles above 65°. ( c ) The effective refractive index profile of the nanopillars changes with the pedestals height which is decreased from 180 to 60 nm. For lower angles, the reflection decreases with the height of the pedestals. For larger angles (>60°), however, the anti-reflection is slightly better for smaller pedestals. Full size image To conclude, we experimentally demonstrated and theoretically modelled the broadband, omnidirectional anti-reflection properties of the transparent glasswings. Our optical analysis showed that the omni-directionality is caused by the random height distribution of the nanopillars. By optimizing the variance of the distribution and the shape of the pedestals, almost perfect anti-reflection surfaces can be engineered for a broadband range of wavelengths and a wide range of viewing angles. Such anti-reflective surfaces could be adapted to improve the light collection in solar cells or for an efficient light extraction of the substrate modes in light-emitting diodes or even enhancing the performance of the optical, optoelectronic and electro-optical devices, such as glasses, mirrors, lens, photodetectors, surface-emitting lasers, displays and optical sensing or imaging [20] , [21] , [30] , [31] , [32] . The large-scale fabrication of the presented random height structures seems feasible. A master mould of these structures can be produced by advanced etching techniques [30] . Moulds replicated from such a master can be used for thermal nanoimprint [33] or hot embossing [34] to replicate glasswing structures on large scales. In comparison with classical multilayer broadband anti-reflection coatings that add up to at least 1 μm thickness to the surface [20] , [35] , the glasswing structures are comparably thin as their mean height is only 500 nm and in addition they are hydrophobic. In fact, engineered glasswing inspired anti-reflective coatings could be thinner than 500 nm if a suitable random height distribution is included into the design. High-resolution imaging Several dried samples of Greta oto were kindly supplied by the Insel Mainau (Insel Mainau, Germany). The butterflies were coated with 15 nm thin gold layer (K575X sputter coater, Quorum Technologies Ltd.) before examination by SEM and FIB (FEI Strata 400S and Zeiss Auriga 60, FEI Company). Topographical analysis ImageJ, a public domain and Java-based image processing programme tool, is used to do the statistical analysis of the nanopillar size on the glasswing membrane. The built-in ‘Analyse’ plugin is applied to perform the histogram analysis of height and radius of every nanopillar analysed. The two-dimensional Fourier power spectrum is obtained out of the SEM picture reported in Fig. 2a , and calculated by using the fast Fourier transform algorithm of Matlab. Optical experimental analysis We measured the reflection spectra on both sides of the glasswings in the visual regime with an ultraviolet–visible Spectrometer Lambda 1050 (PerkinElmer Inc.). An InGaAs 150-mm integrating sphere and a three-detector module were used to measure the diffuse and specular reflection, respectively. Angle-resolved specular reflectivity measurements were carried out using two optical measurement systems. The universal reflectance accessory from PerkinElmer Inc. was used for automated measurements for incidence angles ranging from 8° to 65° and wavelengths from 200 to 800 nm. A stabilized He-Ne laser (632.8 nm) was used to measure reflection up to 80° using a home-built set-up [17] . Here the reflectance is measured through a fibre-coupled USB spectrometer (Ocean Optics HR2000+ with a detection range of 394–840 nm and a resolution of 0.5 nm). The aperture angle was set to 3°. The angle-resolved transmission measurement is carried out with Agilent Cary 5000 ultraviolet–visible–NIR spectrophotometer (Agilent Technologies Inc.). The aperture before the detector, that is, the solid angle was kept to 2° and the integration time for the detector was 2 s. The subsequent data analysis is done with Matlab together with the commercial software package SpectraSuite for data collection from the spectrometer. The optical fibre and the sample holder are rotatable in the x - y plane to measure the specular angle-resolved reflectance spectra. All measurements were taken in the dark to avoid possible stray lights from the surrounding. A reference measurement is done with a mirror and a calibrated commercial spectralon to calculate the relative specular and diffuse reflectance, respectively. Optical simulation method All analytic solutions were calculated with Matlab using the equations given in the text. The developed multilayer thin-film calculator is based on matching the boundary conditions for Maxwells equations. In difference to the Fresnel coefficients that utilizes the total electric and magnetic fields of the waves, only the tangential components are used here to calculate the reflection and transmission coefficient and further the reflectance and transmittance for all incidence angles and both polarizations. Calculations are done first for individual polarizations and by taking the average afterwards to consider the unpolarized light ((TE+TM)/2) condition. To include the absorption of chitin in the calculation, we include the phase components of the fields effectively based on the equations (2.80)–(2.84) from ref. 24 . Correction factors are introduced to take into account all the multiple reflections occurring on the backside of the wing that impact the overall value of the calculated reflection and transmission. The intensity of the light propagating within the wing is attenuated by a factor equal to e − lα , where l is the total distance travelled by the light within the wing (of thickness=550 nm) before escaping into the incident medium and α is the absorption coefficient defined by 4 πκ / λ (with κ being the extinction coefficient and λ is the operational wavelength). The correction factor, calculated for each angle of incidence, is then used by considering an infinite number of reflected and transmitted beams. Please see Supplementary Note 1 for more details. How to cite this article: Siddique, R. H. et al . The role of random nanostructures for the omnidirectional anti-reflection properties of the glasswing butterfly. Nat. Commun. 6:6909 doi: 10.1038/ncomms7909 (2015).